Visualizing active membrane protein complexes by electron cryotomography Unravelling the structural organization of membrane protein machines in their active state and native lipid environment is a major challenge in modern cell biology research. Here we develop the STAMP (Specifically TArgeted Membrane nanoParticle) technique as a strategy to localize protein complexes in situ by electron cryotomography (cryo-ET). STAMP selects active membrane protein complexes and marks them with quantum dots. Taking advantage of new electron detector technology that is currently revolutionizing cryotomography in terms of achievable resolution, this approach enables us to visualize the three-dimensional distribution and organization of protein import sites in mitochondria. We show that import sites cluster together in the vicinity of crista membranes, and we reveal unique details of the mitochondrial protein import machinery in action. STAMP can be used as a tool for site-specific labelling of a multitude of membrane proteins by cryo-ET in the future. The structural and functional organization of biological membranes and their resident protein complexes are of central importance in biomedical research. To date, few tools are available to identify molecular machines within their native lipid environment and to study their dynamic distribution on the nanometre scale. Electron cryotomography (cryo-ET) bridges the gap between light microscopy, which provides low-resolution information and high-resolution protein structures determined by X-ray crystallography. One advantage of cryo-ET over conventional electron microscopy (EM) is the ability to visualize proteins within whole cells or organelles (<500 nm), without staining or dehydration of the sample, reducing the risk of artefacts. However, it is a major challenge to localize specific cellular components in the complex overcrowded milieu of the cell. In principle, clonable heavy metal tags such as bacterial ferritin [1] or concatenated metallothioneins [2] can be used as labels in cryo-ET. Ferritin has a dense iron core (capable of binding up to 4,500 Fe(III) atoms) [3] and low cytotoxicity, and is visible in tomograms as a large ~450 kDa multisubunit assembly [1] . However, because it is an oligomer, multiple copies of a cloned target protein assemble onto one ferritin complex [1] , which carries the risk of mislocalization and likely restricts its use to soluble proteins. Metallothioneins are heavy metal binding proteins of ~6 kDa, and may be used in tandem copies if required. The heavy metal clusters (for example, Pt, Au, Cd) are small (typically <40 metal atoms per metallothionein) [4] and therefore, more difficult to detect in noisy tomographic volumes. Their use has so far been limited to well-characterized soluble proteins, which are present in high copy numbers [5] , [6] , so that the extra density provided by the metal cluster is easily apparent. It seems unlikely that metallothionein tags will be suitable for many in vivo studies, as the production of the protein is dependent on growth of cells in high concentrations of reactive and often cytotoxic heavy metal ions. Such tags are likely to prove their worth in identification of oligomers, or of subunits within large complexes after subtomogram averaging. Other clonable tags with potential importance for correlative light and EM include the fluorescent labels FlAsH and ReAsH [7] , [8] . The site of the fluorescent signal is seen in the electron microscope as a photo-oxidized precipitate. However, cells must be treated with antidotes to prevent cytotoxicity [8] , and moreover in electron cryomicroscopy (cryo-EM), interesting structural detail would be obscured by the large size of the deposit [9] . The discrimination between active and inactive populations of membrane protein complexes by cryo-ET has been largely intractable. Recent advances in correlative light and EM [7] , such as the development of quantum dots (QDs), have opened up new perspectives to overcome these problems. QDs are brightly fluorescent and directly visible in the electron microscope due to their high electron scattering potential, containing between 100 and 100,000 Cd and Se atoms [10] . However, the few published cryo-EM studies have relied on antibody-QD labelling in fixed and stained material [11] , [12] , which limits resolution and identification of proteins. Here we describe a novel approach to labelling for cryo-ET, called STAMP (Specifically TArgeted Membrane nanoParticle), which overcomes many of the drawbacks associated with currently available heavy metal tags. To demonstrate this, we compare our labelling method with the previously reported metallothionein technology [2] , [5] , [6] . We have used STAMP to visualize a membrane-bound molecular machine in action, without the need for compromising fixatives or stains. In order to specifically select for the active complexes, we use a three-step labelling process: (1) production of a small, tagged ligand; (2) specific targeting to active membrane complexes; (3) attachment of dense QD nanoparticles. Mitochondria have an outer and an inner membrane and contain at least 1,000 different proteins synthesized in the cytosol. The majority of these proteins contain amino-terminal targeting signals (presequences) and are destined for the mitochondrial inner membrane or matrix. Concomitant import of these preproteins by the general translocase of the outer membrane (TOM complex) and the presequence translocase of the inner membrane (TIM23 complex) leads to the formation of translocation intermediates that span both membranes [13] , [14] , [15] . The analysis of these translocation contact sites between mitochondrial outer and inner membranes has been difficult, as their visualization has so far only been possible at low resolution in chemically fixed and sectioned samples [16] , [17] . Thus, only limited information is available on the structural organization and spatial distribution of these intricate protein-trafficking molecular hubs. Using STAMP, the three-dimensional distribution and organization of protein import sites in mitochondria is demonstrated. Importing protein complexes are located in discrete clusters, close to, but not directly at crista junctions (CJs). Detailed analysis of the preprotein import machinery in action reveals that the TOM–TIM23 supercomplex is tethered by protein–protein interactions and does not involve close membrane contacts [16] , [17] . Labelled proteins arrest as membrane spanning intermediates We devised a protocol for the site-specific QD labelling of a recombinant model preprotein that can be quantitatively arrested as a two-membrane spanning translocation intermediate ( Fig. 1a ). Model preproteins consisting of N-terminal parts of cytochrome b 2 fused to dihydrofolate reductase (DHFR) have been widely used for biochemical studies on the import reaction. We generated a variant of cytochrome b 2 Δ-DHFR [18] containing a unique carboxy-terminal cysteine residue ( Fig. 1b ), which is indistinguishable from the unmodified model preprotein in terms of import and arrest ( Supplementary Fig. 1 ). On expression and purification of b 2 Δ-DHFR cys from Escherichia coli , a biotin label was attached to the C-terminal cysteine ( Supplementary Fig. 2a,b ). Saturating amounts of the preprotein b 2 Δ-DHFR biotin were incubated with isolated yeast mitochondria in the presence of methotrexate (MTX). MTX stabilizes the folded state of DHFR, and therefore b 2 Δ-DHFR biotin accumulates as an arrested preprotein in TOM–TIM23 import sites ( Fig. 1c ). The biotinylated moiety remains on the outer mitochondrial surface for subsequent labelling, and was fully accessible to streptavidin binding ( Supplementary Fig. 2c ). We then attached biocompatible streptavidin-QD 525 to the biotin-tag on the accumulated preprotein to mark active import sites in mitochondrial samples ( Supplementary Note 1 ). Excess QDs were removed by OptiPrep gradient centrifugation, whereby in the presence of accumulated preproteins, fluorescent QD 525 labelling of mitochondria was observed ( Fig. 1d ). The labelled mitochondrial fractions and unlabelled control mitochondria were recovered from the gradients and analysed by cryo-ET. 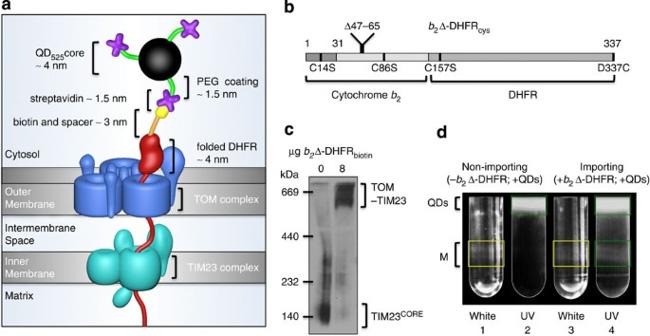Figure 1: Design and implementation of the approach. (a) Schematic of the STAMP (Specifically TArgeted Membrane nanoParticle) approach. In the first step, a small biotin label (yellow) is attached via a spacer arm (orange) to a mitochondrial model preprotein (red). Subsequently, the labelled preprotein is targeted to the mitochondrial import machinery and arrested by means of a tightly folded DHFR domain as a translocation intermediate spanning both TOM (blue) and TIM23 (cyan) complexes. In the third step, the DHFR-linked biotin is bound by streptavidin (purple)-conjugated QDs (black sphere with green spacer arms). The total distance from the QD to the outer mitochondrial membrane is ~10 nm. (b) The design of the mitochondrial model preprotein is based on the fusion proteinb2Δ-DHFR18. To enable site-specific biotinylation, endogenous cysteines (C14, C86 and C157) were substituted with serine and a unique cysteine replaced the C-terminal residue D337. (c) Blue native electrophoresis and western blot analysis of the preprotein-tethered TOM–TIM23 supercomplex detected with an antibody against Tim23. Note that the TIM23 core complexes (TIM23CORE) are quantitatively shifted into TOM–TIM23 supercomplexes on addition ofb2Δ-DHFRbiotin, indicating that the import sites are occupied by preproteins under these conditions. The experiment was repeated three times. (d) Free QDs were separated from labelled mitochondria on an OptiPrep gradient. Under white light (tubes 1 and 3) mitochondrial membranes are visible (M, yellow boxes), and under UV excitation, QD525is detected (tubes 2 and 4; green boxes). QD525co-localization with mitochondria is seen in tube 4. Figure 1: Design and implementation of the approach. ( a ) Schematic of the STAMP (Specifically TArgeted Membrane nanoParticle) approach. In the first step, a small biotin label (yellow) is attached via a spacer arm (orange) to a mitochondrial model preprotein (red). Subsequently, the labelled preprotein is targeted to the mitochondrial import machinery and arrested by means of a tightly folded DHFR domain as a translocation intermediate spanning both TOM (blue) and TIM23 (cyan) complexes. In the third step, the DHFR-linked biotin is bound by streptavidin (purple)-conjugated QDs (black sphere with green spacer arms). The total distance from the QD to the outer mitochondrial membrane is ~10 nm. ( b ) The design of the mitochondrial model preprotein is based on the fusion protein b 2 Δ-DHFR [18] . To enable site-specific biotinylation, endogenous cysteines (C14, C86 and C157) were substituted with serine and a unique cysteine replaced the C-terminal residue D337. ( c ) Blue native electrophoresis and western blot analysis of the preprotein-tethered TOM–TIM23 supercomplex detected with an antibody against Tim23. Note that the TIM23 core complexes (TIM23 CORE ) are quantitatively shifted into TOM–TIM23 supercomplexes on addition of b 2 Δ-DHFR biotin , indicating that the import sites are occupied by preproteins under these conditions. The experiment was repeated three times. ( d ) Free QDs were separated from labelled mitochondria on an OptiPrep gradient. Under white light (tubes 1 and 3) mitochondrial membranes are visible (M, yellow boxes), and under UV excitation, QD 525 is detected (tubes 2 and 4; green boxes). QD 525 co-localization with mitochondria is seen in tube 4. Full size image As a comparison with STAMP, we also engineered both two and three tandem copies of the metallothionein protein to cytochrome b 2 Δ-DHFR ( b 2 Δ-DHFR-MT2 and b 2 Δ-DHFR-MT3, respectively). b 2 Δ-DHFR-MT3 was found to express poorly as aggregates in all E. coli strains, at various temperature, induction conditions and metal (Au/Cd/Zn) conditions tested, thus was not pursued further. b 2 Δ-DHFR-MT2 could be expressed and purified at low amounts (60 μg l −1 cell culture compared with 4 mg l −1 for b 2 Δ-DHFR cys ) in cells supplemented with Au + ( Supplementary Fig. 3a ). On in vitro import of radiolabelled b 2 Δ-DHFR-MT2, the TOM–TIM23 supercomplex was formed in the presence of MTX ( Supplementary Fig. 3b ). In contrast to unmodified b 2 Δ-DHFR or b 2 Δ-DHFR cys , a substantial fraction of b 2 Δ-DHFR-MT2 also accumulated in TOM–TIM23 supercomplexes in the absence of MTX, and thus independently of the folding state of DHFR ( Supplementary Fig. 3b ). We conclude that the fused MT2 itself inhibits the full translocation of preprotein into the mitochondrial matrix. Incubation of the expressed and purified preprotein with isolated mitochondria resulted in efficient b 2 Δ-DHFR- MT2 (Au + ) accumulation as a TOM–TIM23 supercomplex intermediate ( Supplementary Fig. 3c ). Visualization of active preprotein import sites in situ In tomograms of b 2 Δ-DHFR biotin -loaded mitochondria, the distribution of active import sites was visualized via the specifically attached QD 525 with excellent spatial resolution ( Fig. 2a,b , Supplementary Movie 1 ). Import sites were found around the entire circumference of mitochondria, yet their distribution appeared non-uniform and clustered. Close inspection of a large mitochondrial import site cluster revealed that it was located in the vicinity of, but not directly apposed to the CJ ( Fig. 1c ), which connects crista membranes to the inner boundary membrane [19] , [20] . 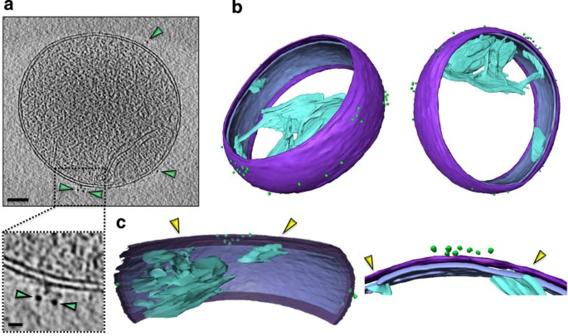Figure 2: Preprotein import sites are non-uniform. (a) A slice through a tomogram reveals the location of QDs (green arrowheads); scale bar, 100 nm, inset=10 nm. (b) Segmentation of the volume shows the distribution of QDs (green spheres) around the mitochondrion. The outer membrane (purple), the inner membrane (lilac) and the crista membranes (cyan) are also shown. (c) Close-ups of the import sites reveal the position of clusters relative to mitochondrial membranes and CJs (yellow arrowheads). Figure 2: Preprotein import sites are non-uniform. ( a ) A slice through a tomogram reveals the location of QDs (green arrowheads); scale bar, 100 nm, inset=10 nm. ( b ) Segmentation of the volume shows the distribution of QDs (green spheres) around the mitochondrion. The outer membrane (purple), the inner membrane (lilac) and the crista membranes (cyan) are also shown. ( c ) Close-ups of the import sites reveal the position of clusters relative to mitochondrial membranes and CJs (yellow arrowheads). Full size image Analysis of tomograms of mitochondria loaded with b 2 Δ-DHFR- MT2 (Au + ) did not enable the location of import sites to be determined. Mitochondria with arrested preprotein showed dark spots on the outer membrane ( Supplementary Fig. 3e ), which were comparable in size to the observed densities of b 2 Δ-DHFR- MT2 (Au + ) alone in solution (~3 nm, Supplementary Fig. 3d ). However, after analysis of control tomograms of non-importing mitochondria ( Supplementary Fig. 3f ), it was apparent that the metallothionein tag could not be distinguished from protein densities on the outer surface of mitochondria. Labelling using metallothionein was therefore not continued further. Determining the specificity of STAMP The limitation of tomographic tilt angles (±~60°) results in a missing wedge of information [21] . This is centred around the z -axis in Fourier space, so that mitochondrial membranes that run parallel to the grid plane are poorly defined in the tomographic reconstruction. While QD 525 -labelled import sites were easily distinguished on membranes perpendicular to the grid plane, they were only visualized with confidence on all surfaces in a few cases ( Table 1 ). This is due to the relatively small size of QD 525 (4 nm spherical core). To resolve this problem, we used QD 605 (4 × 9.4 nm ellipsoidal core), which is larger and more easily visible by EM ( Supplementary Fig. 4b–d ). Moreover, the brighter red fluorescence of QD 605 is complementary to MitoTracker Green, which stains mitochondria regardless of membrane potential, allowing us to reliably determine the specificity of our labelling technique by fluorescence microscopy. In this way, statistical information on the specificity of QD 605 labelling could be collected from a much larger sample size, thus counteracting the common issue of small sample sizes obtained by cryo-ET. After QD 605 incubation and density gradient separation ( Fig. 3a ), the preprotein-loaded mitochondria were labelled, demonstrating that the mitochondria used in our assays were import competent ( Fig. 3b , Supplementary Fig. 5 ). The distribution of QDs on mitochondria was uneven, in agreement with tomographic data. Seven percent of QD 605 fluorescence did not co-localize with mitochondria, which may be due to the disruption of some organelles during sample preparation, giving rise to membrane fragments that still contain bound QD 605 -labelled preproteins. In contrast, 99.7% of control mitochondria that were not preloaded with preproteins did not show QD 605 labelling under the same conditions, indicating an extremely low interference from nonspecifically associated QDs, also in agreement with tomographic data ( Supplementary Movie 2 ). Table 1 Number of QD 525 -labelled import sites per mitochondrion. 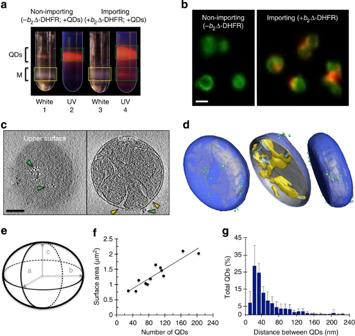Figure 3: Specific labelling determines the total number of preprotein import sites and the degree of clustering. (a) Free QDs were separated from labelled mitochondria on an OptiPrep gradient. Under white light (tubes 1 and 3) mitochondria are visible (M, yellow boxes), and under UV excitation, QD605is detected (tubes 2 and 4; green boxes). QD605co-localization with mitochondria is seen in tube 4. The experiment was repeated four times. (b) Confocal fluorescence images of non-importing and importing mitochondria. The mitochondria are labelled with MitoTracker Green and QD605fluorescence is shown in red; scale bar, 1 μm. The black space between mitochondria has been removed (original inSupplementary Fig. 5a). The statistics described in the text were calculated based onn=350 for the control andn=140 for the actively importing mitochondria. (c) A slice near the top of the tomogram reveals the location of a cluster of QDs (green arrowheads) on the mitochondrial surface. A slice through the centre shows the position of the cluster with respect to the CJs (yellow arrowheads); scale bar, 100 nm, cluster measures ~80 × 60 nm. (d) Segmentation of the volume depicts the three-dimensional distribution of QDs (green spheres) around the mitochondrion relative to the outer membrane (blue) and the cristae (yellow). (e) A model of an ellipsoid was used to calculate the surface area of mitochondria based ona,bandcradii as depicted. (f) A line graph shows the correlation between mitochondrial size and the number of preprotein import sites,n=12 mitochondria as seen inTable 2. (g) Averaged histogram showing the closest distance between two QDs, calculated from 12 mitochondrial samples (Supplementary Fig. 6) accumulating 1,159 QD605data points in total. Error bars indicate the s.d. of the frequency distribution for each minimal distance. Full size table Figure 3: Specific labelling determines the total number of preprotein import sites and the degree of clustering. ( a ) Free QDs were separated from labelled mitochondria on an OptiPrep gradient. Under white light (tubes 1 and 3) mitochondria are visible (M, yellow boxes), and under UV excitation, QD 605 is detected (tubes 2 and 4; green boxes). QD 605 co-localization with mitochondria is seen in tube 4. The experiment was repeated four times. ( b ) Confocal fluorescence images of non-importing and importing mitochondria. The mitochondria are labelled with MitoTracker Green and QD 605 fluorescence is shown in red; scale bar, 1 μm. The black space between mitochondria has been removed (original in Supplementary Fig. 5a ). The statistics described in the text were calculated based on n =350 for the control and n =140 for the actively importing mitochondria. ( c ) A slice near the top of the tomogram reveals the location of a cluster of QDs (green arrowheads) on the mitochondrial surface. A slice through the centre shows the position of the cluster with respect to the CJs (yellow arrowheads); scale bar, 100 nm, cluster measures ~80 × 60 nm. ( d ) Segmentation of the volume depicts the three-dimensional distribution of QDs (green spheres) around the mitochondrion relative to the outer membrane (blue) and the cristae (yellow). ( e ) A model of an ellipsoid was used to calculate the surface area of mitochondria based on a , b and c radii as depicted. ( f ) A line graph shows the correlation between mitochondrial size and the number of preprotein import sites, n =12 mitochondria as seen in Table 2 . ( g ) Averaged histogram showing the closest distance between two QDs, calculated from 12 mitochondrial samples ( Supplementary Fig. 6 ) accumulating 1,159 QD 605 data points in total. Error bars indicate the s.d. of the frequency distribution for each minimal distance. Full size image Calculation of the number of preprotein import sites Cryo-ET analysis of mitochondria labelled with arrested preproteins and QD 605 provided a clear three-dimensional view of active import sites in 12 different mitochondrial samples ( Fig. 3c,d , Table 2 , Supplementary Movie 3 ). For statistical analysis, we collected tomograms of ellipsoidal mitochondria to reveal a linear correlation between the mitochondrial surface area (equation (1), Methods) and the number of QDs, with an average value of 69 QD 605 -labelled active import sites per μm 2 ( Fig. 3e,f , Table 2 ). Calculations performed with the data set obtained with QD 525 ( Table 1 ) revealed an average value of 66 QD 525 -labelled active import sites per μm 2 , demonstrating that QD size was not limiting for the quantitative labelling of import sites. Table 2 Number of QD 605 -labelled import sites per mitochondrion and the percentage found in clusters. Full size table Labelling with QD 605 enabled us to investigate the non-uniform distribution of import sites in detail on a larger data set. The distance between QD neighbours was calculated for each mitochondrion ( Supplementary Fig. 6 ), revealing a clear trend for import sites to be located ~30 nm apart ( Fig. 3g ). On average, 67% of import supercomplexes were seen in distinct clusters of two or more QDs located <50 nm apart ( Fig. 3g , Table 2 ). Preprotein import occurs at specific microdomains We occasionally observed mitochondrial fusion intermediates with two adjacent, but separate inner membranes surround by one single outer membrane [22] ( Fig. 4a , Supplementary Fig. 7 and Supplementary Movie 4 ). Interestingly, analysis of an importing mitochondrion with this feature revealed a marked increase (25% of the mitochondrion total) of QD 605 -labelled import sites in the vicinity of the two tightly aligned inner membranes, indicative of focused targeting to specific membrane regions. 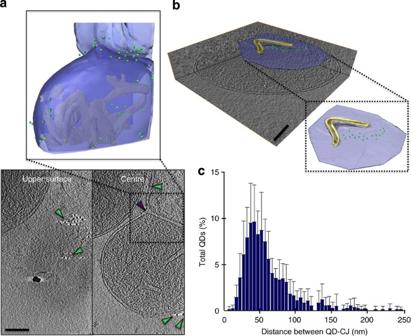Figure 4: Preprotein import occurs at discrete microdomains. (a) A slice near the top of a tomogram reveals the location of clusters of QDs (green arrowheads) on the mitochondrial surface. A slice through the centre shows further QDs and the fusion septum (purple arrowhead); scale bar, 100 nm, cluster measures ~150 × 60 nm. Segmentation of the volume depicts the three-dimensional distribution of QDs (green spheres) around the mitochondrion with respect to the cristae (yellow) and around the mitochondrial septum. The outer membrane is rendered in two colours (light and dark blue) in order to distinguish the position of the septal ring. (b) Partial segmentation of the upper surface of a mitochondrion reveals the position of QDs (green spheres) with respect to a slit-like CJ (yellow) on the inner boundary membrane (mauve). For clarity, the outer membrane is not shown; scale bar, 100 nm, cluster measures ~50 × 250 nm. (c) Averaged histogram showing the closest distance between QD and CJs, calculated from nine mitochondrial samples (Supplementary Fig. 8) accumulating 836 QD605data points in total. Error bars indicate the s.d. of the frequency distribution for each minimal distance. Figure 4: Preprotein import occurs at discrete microdomains. ( a ) A slice near the top of a tomogram reveals the location of clusters of QDs (green arrowheads) on the mitochondrial surface. A slice through the centre shows further QDs and the fusion septum (purple arrowhead); scale bar, 100 nm, cluster measures ~150 × 60 nm. Segmentation of the volume depicts the three-dimensional distribution of QDs (green spheres) around the mitochondrion with respect to the cristae (yellow) and around the mitochondrial septum. The outer membrane is rendered in two colours (light and dark blue) in order to distinguish the position of the septal ring. ( b ) Partial segmentation of the upper surface of a mitochondrion reveals the position of QDs (green spheres) with respect to a slit-like CJ (yellow) on the inner boundary membrane (mauve). For clarity, the outer membrane is not shown; scale bar, 100 nm, cluster measures ~50 × 250 nm. ( c ) Averaged histogram showing the closest distance between QD and CJs, calculated from nine mitochondrial samples ( Supplementary Fig. 8 ) accumulating 836 QD 605 data points in total. Error bars indicate the s.d. of the frequency distribution for each minimal distance. Full size image Our results with QD 525 furthermore indicated a spatial correlation between import sites and CJs ( Fig. 2c ). QD 605 labelling of a mitochondrion with a long slit-like CJ on the upper surface revealed a large cluster of import sites located directly between the two branches of the junction ( Fig. 4b ). To investigate the spatial relationship between import sites and CJs in detail, we calculated the distances from QD 605 to the closest CJ in nine different mitochondrial samples ( Supplementary Fig. 8 ). This revealed that rather than directly neighbouring CJs, import sites tend to be located 30–60 nm away on average ( Fig. 4c ). Structural insights into the import supercomplex Apart from showing the relative distribution of active preprotein import sites, our results also provide the first insights into their structural organization at the macromolecular level. Earlier studies of chemically fixed samples proposed a closer proximity of mitochondrial outer and inner membranes at translocation contact sites [16] , [17] . Our tomograms of unfixed and unstained mitochondria collected with a K2 direct electron detection camera now uncover unprecedented details of the two-membrane spanning translocation intermediates ( Fig. 5 , Supplementary Movie 5 ). First, there is no measurable difference in the distance between both lipid bilayers at active import sites compared with other regions away from the positions of QD labelling ( Fig. 5 , Table 3 ). Second, we observe distinct protein densities protruding from the outer membrane and spanning the intermembrane space ( Fig. 5 ). To examine these more closely, all data collected under identical conditions were combined, which revealed that the outer membrane protein density located directly beneath the QD was well conserved in 91% of cases. The intermembrane space spanning protein density was in turn clearly determined in 96% of cases. These data were then subject to subtomogram averaging, which revealed the overall shape of conserved protein densities at the sites of QD labelling, that likely represent parts of the active protein import machinery ( Supplementary Fig. 9 ). 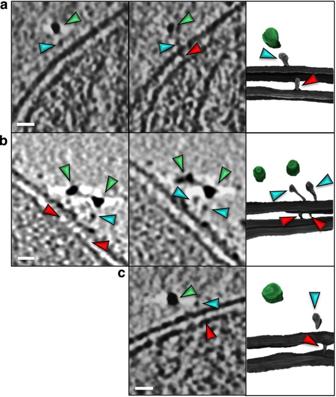Figure 5: Details of the import supercomplex. Left panels: close inspection of the protein densities localized 10 nm beneath the QDs (green arrowheads) reveals characteristic features on the outer membrane (blue arrowheads) and protein densities spanning the intermembrane space (red arrowheads). The multiple panels inaandbrepresent different slices through the same tomogram; incall features were visible in one slice; scale bars, 10 nm. Right panels: the segmented volumes of the same features in three dimensions (QDs green). Figure 5: Details of the import supercomplex. Left panels: close inspection of the protein densities localized 10 nm beneath the QDs (green arrowheads) reveals characteristic features on the outer membrane (blue arrowheads) and protein densities spanning the intermembrane space (red arrowheads). The multiple panels in a and b represent different slices through the same tomogram; in c all features were visible in one slice; scale bars, 10 nm. Right panels: the segmented volumes of the same features in three dimensions (QDs green). Full size image Table 3 Distance across the intermembrane space. Full size table The study of active biological machines in their native environment is a major new field of scientific discovery. To pinpoint proteins of interest, it is paramount to develop specific labels that are small enough not to compromise biological function, yet are large enough to be distinguished. Our new STAMP (Specifically TArgeted Membrane nanoParticle) approach constitutes an elegant means to specifically select for protein complexes in situ . In particular, STAMP is widely applicable for the localization of ligand-binding membrane protein complexes in their active states. It consists of three consecutive steps: (1) selective labelling of a ligand with a small non-toxic tag; (2) specific targeting of the labelled ligand to the corresponding membrane protein complex; (3) selective binding of the membrane-targeted ligand by dense QD nanoparticles. We have used this approach in the study of mitochondrial preprotein import complexes, and compared it with the previously reported metallothionein tag [2] , [5] , [6] . The added density in b 2 Δ-DHFR- MT2 (Au + ) was visualized in tomograms of the protein alone in solution, but on arrest across the TOM–TIM23 complex could not be distinguished with confidence from proteins bound to the mitochondrial outer membrane. This is due to the small size of the MT tag (~3 nm) compared with QD 525 (~4 nm) or QD 605 (~4 × 9.4 nm), in addition to the reduced electron scattering potential (compare Fig. 3c with Supplementary Fig. 3d ). STAMP has the added benefit of being a multi-purpose tag, both dense and fluorescent, which we have used to full advantage in our studies. Using STAMP, we were able to visualize mitochondrial preprotein import sites, which revealed their non-uniform distribution on the mitochondrial surface. Notably, these data are consonant with super-resolution microscopy analysis of whole cells, which detected clustering of the TOM complex receptor Tom20 in mitochondria [23] . Clusters of Tom20 were determined to be ~30–40 nm in diameter [23] , which is in the same range as data presented here ( Figs 3c and 4a,b ). It should, however, be noted that we report on the localization and organization of active preprotein-carrying TOM–TIM23 supercomplexes, which is not equivalent to the Tom20 receptor in isolation. Moreover, the TOM complex is much more abundant than the TIM23 complex and hands over incoming mitochondrial proteins to several distinct downstream import and sorting pathways. Thus, the mitochondrial TOM complex population likely contains different pools that cooperate with different partner protein complexes [13] , [14] , [15] . We speculate that the local accumulation of TOM–TIM23 import sites may enable focused preprotein targeting to areas within the mitochondria that are in the process of major morphological changes. This idea is in line with the observed accumulation of active import sites in the vicinity of crista membranes, which are highly dynamic structures that undergo extensive remodelling in response to metabolic and developmental cues [20] . Interestingly, CJ proteins, like Mic60 (mitofilin), have been reported to form inner–outer membrane contacts that contain a fraction of TOM complexes [24] . However, these contact sites are thought to be distinct from the translocation contact sites spanned by arrested preproteins [17] . An earlier immunolabelling study did not reveal any particular tendency for Tom20 or Tim23 to locate in the vicinity of CJs [25] . However, this would be difficult to conclude with confidence from two-dimensional projections of chemically fixed and stained sections. The spatial correlation between CJs and preprotein import sites may now encourage a reassessment of the functional relationship between different mitochondrial membrane contact sites. We frequently observed protein densities, both protruding from the outer membrane and spanning the distance across the IMS, at active import sites. The dimensions of the IMS densities suggest more than a single extended translocating polypeptide chain. Suspended between the TOM and TIM23 complexes, the translocated polypeptide thus seems to interact with protective or physically reinforcing proteins to generate the specific molecular architecture of active import sites [26] , [27] . Notably, the observed outer membrane protein density measuring ~10 nm in height has similar dimensions as the cytosolic domain of the Tom70 import receptor as revealed by X-ray crystallography [28] . Further mutational studies and subtomogram averaging based on larger data sets will provide more comprehensive structural information on this dynamic molecular machinery at work. We used a three-step protocol to specifically label the active machinery engaged in mitochondrial preprotein import. Other intracellular protein translocation systems can now be studied with little modifications to our protocol. Moreover, we assume that this approach will also prove particularly informative with respect to the investigation of antigen-binding B- or T-cell receptors on the cell surface, or ligands binding G-protein-coupled receptors. The STAMP method can also be adapted to label endogenously expressed proteins in a two-step approach, by inclusion of a short 15 amino acid biotin acceptor peptide [29] available in a variety of bacterial and eukaryotic vectors (AviTag, Avidity, CO). The AviTag has already shown potential as a protein domain marker in single particle EM studies [30] . Labelling proteins from within the cell remains a challenge, yet QDs that are able to penetrate membranes represent promising options for the future [31] . Using STAMP, purification of tagged cells, organelles or membranes is followed by incubation with dense nanoparticles. Our approach can therefore be adapted as a tool for site-specific labelling of a multitude of membrane or surface-exposed proteins. Cloning of b 2 Δ-DHFR Plasmid p b 2 Δ-DHFR was generated by cloning a fusion gene that encodes the first 167 residues of cytochrome b 2 (with an internal deletion of residues 47–65), N-terminally fused to mouse DHFR, into the pGEM4 vector [18] , [32] (Promega, Madison, USA). Plasmid p b 2 Δ-DHFR cys , encoding a mutated fusion protein that harbours the amino-acid substitutions C14S, C86S, C157S, and D337C was produced using the Quikchange site-directed mutagenesis kit (Agilent Technologies, Santa Clara, USA). Plasmids p b 2 Δ-DHFR-MT2 and p b 2 Δ-DHFR-MT3 were produced by assembly PCR, using the amplified gene products from plasmids p b 2 Δ-DHFR and pMAL-c2x-MT2, or pMAL-c2x-MT3, respectively [2] . For expression in E. coli , DNA fragments encoding b 2 Δ-DHFR cys , b 2 Δ-DHFR-MT2 and b 2 Δ-DHFR-MT3 were used to replace b 2 Δ-DHFR in the polylinker of the expression vector pUHE-73 [32] , yielding plasmids pUHE- b 2 Δ-DHFR cys , pUHE- b 2 Δ-DHFR-MT2 and pUHE- b 2 Δ-DHFR-MT3, respectively. Primer sequences used in all cloning steps are given in Supplementary Table 1 . Isolation and fractionation of mitochondria The Saccharomyces cerevisiae strain YPH499 ( MAT a, ade2-101 , his3-Δ200 , leu2-Δ1 , ura3-52 , trp1-Δ63 , lys2-801 ) [33] was cultured in YPG medium (1% (w/v) yeast extract, 2% (w/v) Bacto-Peptone and 3% (w/v) glycerol) at 30 °C. At mid-logarithmic phase, cells were collected to isolate mitochondria by differential centrifugation [34] . In brief, on enzymatic digestion of the cell wall, cells were mechanically ruptured and cell debris was removed. Mitochondria were pelleted by centrifugation at 10,000 g . The mitochondrial fraction was diluted in SEM buffer (250 mM sucrose, 1 mM EDTA, 10 mM MOPS-KOH, pH 7.2) to a protein concentration of 10 mg ml −1 . Mitochondria aliquots were snap frozen in liquid nitrogen and stored at −80 °C. Expression of b 2 Δ-DHFR and biotinylation of b 2 Δ-DHFR cys The fusion proteins b 2 Δ-DHFR cys and b 2 Δ-DHFR-MT2 were expressed from plasmids pUHE- b 2 Δ-DHFR cys or pUHE- b 2 Δ-DHFR-MT2 in E. coli BMH 71–18 cells (Clontech, CA, USA) by IPTG induction in LB media at mid exponential phase at 15 °C overnight. Cells expressing b 2 Δ-DHFR-MT2 were additionally supplemented with 0.5 mM sodium aurothiomalate. Cells were pelleted and washed in sucrose buffer (20 mM KPi, pH 8, 30% sucrose, 1 mM EDTA, 10 mM DTT, 1 mM phenylmethylsulphonyl fluoride (PMSF)) and resuspended in MOPS buffer (20 mM MOPS pH 8, 1 mM EDTA, 10 mM DTT, 1 mM PMSF, 0.1% Triton X-100). After cell disruption, insoluble material was removed by centrifugation at 22,000 g for 30 min at 4 °C. The soluble protein was purified from the resulting supernatant via a SP-Sepharose high-performance cation exchanger (GE Healthcare, Buckinghamshire, UK) followed by size-exclusion chromatography over a HiLoad Supadex 75 (16/60) column (GE Healthcare). Purified b 2 Δ-DHFR cys was incubated with a 10-fold molar excess of maleimide-PEG 2 -biotin (Pierce, Rockford, USA) overnight at 4 °C, while gently rotating. Unbound label was removed by size-exclusion chromatography using a high-resolution Supadex 75 (10/300) column (GE Healthcare). Protein preparations were analysed by SDS–PAGE and Coomassie blue staining. Full scans of gels are shown in Supplementary Fig. 10 . The degree of biotinylation was calculated to be 1.1±0.24 moles biotin/mole b 2 Δ-DHFR cys using the HABA biotin quantitation kit (Pierce). In vitro import of precursor proteins into mitochondria Radiolabelled b 2 Δ-DHFR, b 2 Δ-DHFR cys and b 2 Δ-DHFR-MT2 fusion proteins were produced using a transcription/translation rabbit reticulocyte lysate kit (GE Healthcare) in the presence of [ 35 S]-methionine (Perkin Elmer, Waltham, USA). In vitro import experiments were performed by adding either the radiolabelled precursor proteins, the recombinant biotinylated b 2 Δ-DHFR cys ( b 2 Δ-DHFR biotin ) or b 2 Δ-DHFR-MT2 to mitochondria in import buffer (10 mM MOPS-KOH, pH 7.2, 3% (w/v) fatty acid-free BSA, 250 mM sucrose, 80 mM KCl, 5 mM MgCl 2 , 2 mM KH 2 PO 4 , 5 mM methionine) in the presence of 2 mM NADH, 2 mM ATP and an ATP regenerating system (5 mM creatine phosphate and 0.1 mg ml −1 creatine kinase). Arrest of precursor proteins at import sites was achieved by adding 5 μM MTX to the import reaction mix. Reactions were stopped by uncoupling the mitochondrial membrane potential (Δψ) with addition of AVO mix (8 μM antimycin A, 1 μM valinomycin and 20 μM oligomycin, final concentrations) and cooling on ice. Unbound precursor proteins were removed by washing mitochondria with SEM buffer. For SDS–PAGE analysis, samples were solubilized in lysis buffer (60 mM Tris–HCl, pH 6.8, 2% (w/v) SDS, 10% (v/v) glycerol, 0.01% (w/v) bromophenol blue, 2 mM PMSF) for 5 min at 95 °C. Proteins were separated on NuPAGE 4–12% Bis-Tris gels (Invitrogen, Carlsbad, USA). For the analysis of translocation intermediates by blue native electrophoresis, preprotein-loaded mitochondria were resuspended in ice-cold solubilization buffer (20 mM Tris–HCl, pH 7.4, 0.1 mM EDTA, 50 mM NaCl, 1% (w/v) digitonin, and 10% (v/v) glycerol) for 15 min on ice. After a clarifying centrifugation step, soluble proteins were mixed with ice-cold blue native loading buffer (100 mM Bis-Tris–HCl pH 7.0, 5% (w/v) Coomassie Brilliant Blue G-250, 500 mM 6-aminocaproic acid) and subjected to electrophoresis on 6–16.5% polyacrylamide blue native gradient gels. Radioactive protein bands were detected by digital autoradiography and images were processed using Multi Gauge software (Fujifilm, Tokyo, Japan). Immunodecoration of western blots was performed with an antiserum against the Tim23 protein [26] . Irrelevant gel lanes were removed by digital image processing. Full scans of key autoradiographs and western blots are shown in Supplementary Fig. 10 . Labelling of arrested supercomplexes with QDs QDs (Invitrogen, Carlsbad, USA) were centrifuged at 5,000 g for 3 min before use and only the supernatant fraction was used. The starting material, supernatant and pellet were assessed by agarose gel electrophoresis (1% agarose in 40 mM Tris pH 8, 20 mM acetic acid, 1 mM EDTA) and EM ( Supplementary Fig. 4 ). Mitochondria with and without arrested b 2 Δ-DHFR biotin were incubated with a 10-fold excess of streptavidin-coated QDs over the molar amount of Tim23 in the mitochondrial sample, for 4 h at 4 °C with gentle shaking. This was calculated according to the experimentally determined amounts of Tim23 per mg of total mitochondrial protein [35] . The efficiency of streptavidin binding to the b 2 Δ-DHFR biotin -carrying TOM–TIM23 supercomplex was assessed by incubation of preprotein-loaded intact mitochondria with the same relative amount of streptavidin as for the streptavidin-QD labelling reactions before blue native electrophoresis and western blotting. Separation of excess QDs was performed with an OptiPrep density gradient (Sigma-Aldrich, St. Louis, USA), using gradients with 10 steps of 200 μl each, ranging from 0 to 27% iodixanol in ultra-clear centrifuge tubes (Beckman Coulter, Pasadena, USA). Samples were centrifuged at 80,000 g for 20 min at 4 °C with gentle braking. A quantity of 400 μl fractions corresponding to the mitochondrial bands were removed and diluted into 2 ml SEM buffer to dilute OptiPrep medium. Mitochondria were pelleted at 20,000 g for 10 min at 4 °C and resuspended in SEM buffer at a protein concentration of ~10 mg ml −1 . Electron microscopy QD 525 or QD 605 (20 nM) were applied to glow-discharged Cu 400 mesh (Plano, Wetzlar, Germany) continuous carbon-coated support grids and stained with 1% uranyl acetate. Electron micrographs were collected at a magnification of × 45,000 or × 56,000 (corresponding to a pixel size of 0.27 and 0.24 nm, respectively), at 8 μm defocus on a Tecnai Spirit microscope (FEI, Hillsboro, USA), operating at 120 keV and fitted with a 4k × 4k Ultrascan CCD camera (Gatan, Pleasanton, USA). Electron cryotomography Mitochondria at 5 mg ml −1 total mitochondrial protein concentration were mixed 1:1 with 10 nm protein A-gold (Aurion, Wageningen, The Netherlands) as fiducial markers and applied to glow-discharged R2/2 Cu 300 mesh holey carbon-coated support grids (Quantifoil, Jena, Germany). The samples were blotted for ~4 s in a humidified atmosphere and plunge frozen into liquid ethane in a home-made plunge freezing device (Deryck Mills, MPI for Biophysics, Frankfurt). Grids were maintained under liquid nitrogen and transferred into the electron microscope at cryogenic temperatures. Tomograms were collected at tilt steps of 1–2° and 8 μm defocus, using either a Tecnai Polara or Titan Krios microscope (FEI), both equipped with field emission guns operating at 300 keV and Quantum energy filters (Gatan, Pleasanton, USA) operated with slit widths of 20 eV. The Polara is fitted with a 4k × 4k Ultrascan CCD camera and the Krios with a K2 Summit direct electron detection camera (Gatan, Pleasanton, USA). The total dose per image was ~2e − Å −2 for the CCD camera and 8e − per pixel per second for the K2 camera. Tomograms were aligned using the gold fiducial markers and volumes reconstructed by weighted back projection using the IMOD software [36] (Boulder Laboratory, Boulder, USA). Contrast was enhanced by nonlinear anisotropic diffusion (NAD) filtering in IMOD [37] . Segmentation was performed using AMIRA (FEI). The tomographic slice shown in Fig. 2a was collected on the Krios microscope at a magnification of × 26,000 (corresponding to a pixel size of 0.53 nm). Slices shown in Figs 4 were collected on the same microscope at a magnification of × 42,000 (corresponding to a pixel size of 0.33 nm). The tomographic slices shown in Fig. 3c and Supplementary Fig. 3d,f were collected on the Polara microscope at a magnification of × 34,000 (corresponding to a pixel size of 0.6 nm). Calculation of closest QD–QD and QD–CJ distances Clusters were initially visually inspected and it was determined that they occur in groups of QDs 50 nm apart or less (centre-to-centre). A MATLAB (Mathworks, CA, USA) script was developed to accurately measure the distances between QDs and between QDs and CJs. The coordinates of QDs and CJs marked in IMOD were automatically loaded into MATLAB and the distances calculated in an iterative for-loop by Pythagoras theorem. The analysis was repeated for 12 data sets (12 mitochondria from 12 tomograms, accumulating 1,159 QD data points) to extract the minimal QD–QD distances. Of these 12, the 9 mitochondria with the clearest resolved cristae were used for the QD–CJ analysis (accumulating 836 QD data points). Averaged histograms were subsequently calculated, showing the mean frequency of occurrence for each minimal distance between QD–QD and QD–CJ. To account for the different numbers of QDs in each data set, the mean frequency was calculated as a percentage. Calculation of the surface area of a mitochondrion In order to calculate mitochondrial surface area, 17 tomograms were collected of approximately ellipsoidal mitochondria of various sizes, which were labelled with QDs. The surface area of the ellipsoid was calculated from: where a , b and c are the radii along the x , y and z axes of the ellipsoid, respectively (as depicted in Fig. 3e ), and p is a constant 1.6075 (ref. 38 ). Subtomogram averaging Conserved outer membrane and IMS protein densities are only clearly visible on membranes running parallel to the grid plane. The number of particles available for averaging per tomogram is therefore low. Thus, in order to calculate a preliminary model of the QD-marked supercomplex, data from multiple tomograms were combined. Subvolumes marked by 81 QDs from six twice-binned (pixel size=0.66 nm) and NAD contrast-enhanced tomograms, collected at a magnification of × 42,000 at 8 μm defocus with the K2 camera, were averaged using PEET [39] (IMOD software, Boulder Laboratory). Subtomogram averages were calculated independently for the outer membrane and inner membrane space protein densities, then were subsequently combined into a composite model. Three-dimensional maps were analysed and displayed using Chimera (UCSF, San Francisco, USA). The resolution of the average is less than 4 nm, considering that the first zero of the contrast transfer function at the imaging conditions used is at ~3.9 nm, and that the tomograms were contrast enhanced by NAD. Confocal microscopy Mitochondria at a concentration of 1 mg ml −1 total protein concentration were incubated with 50 nM MitoTracker Green (Invitrogen, Carlsbad, USA) for 15 min at 37 °C. A volume of 100 μl of sample was added to individual wells of 8-well chamber slides (Sarstedt, Nümbrecht, Germany) and 200 μl of 1–2% SeaKem low-melting point agarose (Lonza, Basel, Switzerland) dissolved in SEM buffer was added on top to prevent mitochondrial movement. Images were acquired at a magnification of × 63 using an inverted confocal microscope (LSM 710-plan apochromat /1.20 NA/ oil immersion; Carl Zeiss, Jena, Germany) and the ZEN2008 software (Carl Zeiss, Jena, Germany). The excitation laser wavelength was 488 nm and the emission windows were set at 492–535 nm for the MitoTracker Green and 597–700 nm for the QD 605 . The pinhole was set at 1 AU plus a master gain of 750. How to cite this article : Gold, V. A. M. et al. Visualizing active membrane protein complexes by electron cryotomography. Nat. Commun. 5:4129 doi: 10.1038/ncomms5129 (2014).